Roles of dental development and adaptation in rodent evolution In paleontology, many changes affecting morphology, such as tooth shape in mammals, are interpreted as ecological adaptations that reflect important selective events. Despite continuing studies, the identification of the genetic bases and key ecological drivers of specific mammalian dental morphologies remains elusive. Here we focus on the genetic and functional bases of stephanodonty, a pattern characterized by longitudinal crests on molars that arose in parallel during the diversification of murine rodents. We find that overexpression of Eda or Edar is sufficient to produce the longitudinal crests defining stephanodonty in transgenic laboratory mice. Whereas our dental microwear analyses show that stephanodonty likely represents an adaptation to highly fibrous diet, the initial and parallel appearance of stephanodonty may have been facilitated by developmental processes, without being necessarily under positive selection. This study demonstrates how combining development and function can help to evaluate adaptive scenarios in the evolution of new morphologies. Over the past 200 My, the diversification of the masticatory apparatus in mammals has facilitated exploitation of a wider range of foods than in their ancestors [1] , including more plant material. In this evolutionary process, mammals have acquired more heterogeneous dentitions, including fewer but more complex teeth [2] . Today, murine rodents, the Old World mice and rats, are one of the most successful living examples of mammalian radiation, which can partly be explained by the evolution of novel dental morphologies contributing to the colonization of numerous environments and habitats. Although possessing only one ever-growing incisor and three molars per dental quadrant, murines have one of the most derived mammalian dental patterns, typically characterized by numerous cusps arranged in transverse chevrons [3] . Although most murine rodents have omnivorous feeding habits [4] , less than a quarter of species have developed distinct dental adaptations for plant consumption, such as enlarged, complex or high-crowned teeth [5] , [6] , [7] . The fossil record of murine rodents is essential for providing a broad spectrum of pre-existing dental phenotypes. It is also important for documenting successive morphological changes in a temporal framework in relation to feeding adaptations. As understanding the developmental bases of ecologically relevant features is useful in evaluating the adaptive significance of parallel acquisition of similar dental features, both paleontological and developmental data have to be considered in such evolutionary contexts. Stephanodonty is a dental innovation arising independently in more than ten lineages of European and African murine rodents during the last 10 My [8] . The key characteristic of this phenotype was defined as the connection in a garland-like fashion of the five posterior main cusps in first and second upper molars [9] (M 1 –M 2 ). The extinct Stephanomys † genus presents the most advanced stage with the above mentioned garland connected to the anterior chevron via lateral longitudinal crests [8] ( Fig. 1a ). On lower molars (M 1 –M 2 ), the stephanodont pattern corresponds to the occurrence of a single longitudinal central crest. The stephanodont pattern is variable within murine rodents [8] . In the European Stephanomys † lineage, it is weakly expressed in the basal species Progonomys hispanicus † , basic in Occitanomys † , and then fully expressed in Stephanomys † species ( Fig. 1b,c ). In the Apodemus lineage, currently represented by Old World wood and field mice, this pattern is absent in stem species, such as Progonomys cathalai † and Progonomys castilloae † , whereas the garland is present in Apodemus species (for example, Apodemus sylvaticus , Fig. 1b,c ). Such a garland is also present in a few extant and extinct African genera [8] from the Arvicanthini tribe (for example, Paraethomys † , Aethomys , Grammomys , Hybomys , Thallomys and Oenomys , which has a fully expressed stephanodont pattern). 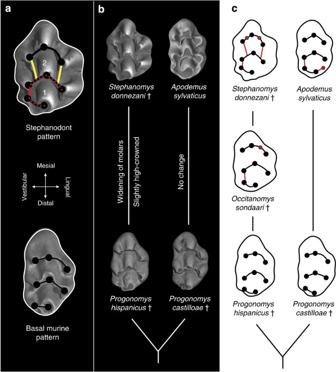Figure 1:Dental morphologies observed inApodemusandStephanomyslineages. (a) Diagrams depicting the stephanodont condition compared with the basal condition. The red dotted line on the diagram indicates the basic stephanodont pattern (1) corresponding to the garland of cusps resulting from the addition of the crest depicted in red colour. Yellow lines represent anterior additional crests indicating the most advanced stage (2). (b) Upper first molars imaged by using X-ray conventional microtomographic three-dimensional renderings. White lines indicate phylogenetic relationships with main dental variations. (c) Dental diagrams showing additional cusps and crests in red dots and red lines, which are characteristic of each species. Dark lines indicate phylogenetic relationships. Not to scale. †: extinct species. Figure 1: Dental morphologies observed in Apodemus and Stephanomys lineages. ( a ) Diagrams depicting the stephanodont condition compared with the basal condition. The red dotted line on the diagram indicates the basic stephanodont pattern (1) corresponding to the garland of cusps resulting from the addition of the crest depicted in red colour. Yellow lines represent anterior additional crests indicating the most advanced stage (2). ( b ) Upper first molars imaged by using X-ray conventional microtomographic three-dimensional renderings. White lines indicate phylogenetic relationships with main dental variations. ( c ) Dental diagrams showing additional cusps and crests in red dots and red lines, which are characteristic of each species. Dark lines indicate phylogenetic relationships. Not to scale. †: extinct species. Full size image Even though this dental pattern has been interpreted as a specialization to an abrasive diet [10] , little is actually known about the factors contributing to the parallel occurrences of stephanodonty over the course of murine evolution, especially the putative function of additional longitudinal crests during food processing. Moreover, the genetic aetiology and the underlying mechanisms involved in the formation of crests remain undescribed, inasmuch as most studies have mainly focused on cusp appearance and development [11] , [12] , [13] , [14] . The ectodysplasin (Eda) signalling pathway is required for normal development of organs of ectodermal origin, such as hair, exocrine glands and teeth [15] , [16] , [17] , [18] . It has been shown that gain or loss of function of implicated genes ( Eda and Edar ) cause defects in the dentition, affecting the size and number of both teeth and cusps [11] , [19] , [20] , [21] . Interestingly, experimental overexpressions of the Eda pathway genes in the laboratory mouse ( Mus musculus ) have previously been described to produce a number of changes in the murine dentition, and longitudinal crests can be observed [11] , [14] , [21] , [22] . Here we compare the dental morphology of Eda and Edar transgenic mice together with those of the well-documented Apodemus and Stephanomys † lineages. These extinct and extant lineages are of interest, as they enable a documentation of the successive stages of stephanodonty through time, as well as the associated variations of crown morphologies. Overexpressing Eda and Edar mice show that the parallel appearance of stephanodonty in different murine lineages may have been facilitated by a relatively simple developmental modification producing longitudinal crests. Using dental microwear analyses, we propose that stephanodonty represents an adaptation to fibrous foods, rather than solely abrasive foods, a dietary shift often related to climatic and environmental changes. However, basic stephanodonty may have been selectively neutral, and only the more advanced stage could have been under positive selection associated with opening up of environments during the Late Miocene. Eda or Edar increase generates stephanodont crests After examination of mice with increased signalling as a result of overexpression of the ligand (K14- Eda ) or carrying a high copy number of its receptor ( Edar Tg951 ), we observe many dental variations compared with wild-type (WT) mice ( Fig. 2 and Supplementary Fig. S1 ). Dental measurements performed on the whole samples showed that homozygous K14- Eda and Edar Tg951/Tg951 generally have shorter molars than controls (except M 1 , Fig. 2 ), and tend to have wider molars (M 1 , M 1 and M 2 ; Supplementary Tables S1 and S2 ). A supernumerary tooth can be frequently observed in front of M 1 (70.4%) in K14- Eda mice and occasionally in front of M 1 (6.9%; Fig. 3 and Supplementary Fig. S1 ). This anomaly is far less frequent in Edar Tg951/Tg951 (3.3% for M 1 and 1.7% for M 1 ) and is absent in heterozygous Edar Tg951 . The length reduction of first molars in these transgenic mice can be explained by the occurrence of vestigial dental buds in front of first molars in mouse [13] , which facilitates the development of a fourth premolar-like tooth, as observed in some mutant mice, especially Eda , Edar and Sprouty 2 losses of function [20] , [23] . 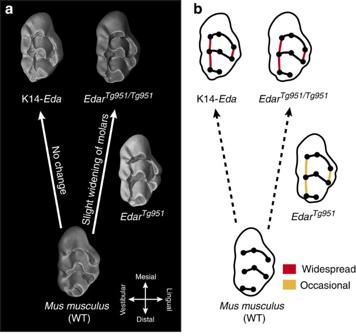Figure 2:Main dental characters observed inEdaandEdartransgenic mice. (a) Upper first molars imaged by using X-ray conventional and synchrotron microtomographic three-dimensional renderings, and main dental variations. (b) Dental diagrams showing additional crests. Colours indicate the frequencies of each morphotype observed: occasional (1–35%), widespread (70–100%). WT, wild type. Figure 2: Main dental characters observed in Eda and Edar transgenic mice. ( a ) Upper first molars imaged by using X-ray conventional and synchrotron microtomographic three-dimensional renderings, and main dental variations. ( b ) Dental diagrams showing additional crests. Colours indicate the frequencies of each morphotype observed: occasional (1–35%), widespread (70–100%). WT, wild type. 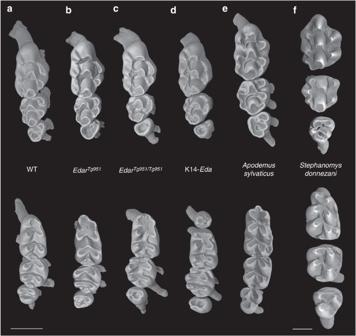Figure 3: Most frequent morphotypes observed in transgenic mice and stephanodont species. (a,c,d) X-ray synchrotron microtomographic three-dimensional renderings of upper and lower cheek tooth rows. (b,e,f) X-ray conventional microtomographic three-dimensional renderings of upper and lower cheek tooth rows. Scale bars, 1 mm. WT, wild type. Full size image Figure 3: Most frequent morphotypes observed in transgenic mice and stephanodont species. ( a , c , d ) X-ray synchrotron microtomographic three-dimensional renderings of upper and lower cheek tooth rows. ( b , e , f ) X-ray conventional microtomographic three-dimensional renderings of upper and lower cheek tooth rows. Scale bars, 1 mm. WT, wild type. Full size image The presence of more or less marked longitudinal crests interconnecting chevrons is unusual in the mouse. Nonetheless, the derived stage involving the garland and the lateral anterior crests occurs in Eda and Edar homozygous transgenic mice ( Fig. 2 ). On lower molars, a central crest, typical of the derived stephanodont pattern, generally appears between chevrons ( Fig. 3 ). As a result, most morphotypes observed in the upper and lower molars of both transgenic animals mirror the canonical features of the derived stephanodont pattern ( Fig. 3 ). However, the posterior insertion of anterior crests is slightly different between transgenic mice and Stephanomys † . In transgenic mice, anterior crests directly link lateral cusps, whereas in Stephanomys † these longitudinal crests are connected to transverse crests. A slight variation is also observed for the central crest in lower molars with a mesial insertion on the vestibular cusp instead of the lingual ( Fig. 3 ). Previous studies on comparable overexpressing transgenic mice also showed that the double transgenic K14- Eda ;K14- Edar displayed a vestibular cingulid (63% of specimens) on lower molars, with a cusp on M 1 (ref. 14 ). These characters are also observed in most stephanodont species ( Fig. 3 ). Dental widening, albeit slight in transgenic mice, is another common trend shared with several extinct stephanodont species ( Figs 1 and 2 , for example, Occitanomys † and Stephanomys † ) even if it is not considered as a general trend, because it does not occur in all species having the garland (for example, Apodemus and Oenomys ). To our knowledge, generation of such longitudinal crests has never been reported in other mutant or transgenic mice. Trends in dental shape related to longitudinal crests Previous studies have shown that variations in dental outline were associated with stephanodonty [24] , [25] , [26] . Using this quantitative method of description of the overall tooth shape, we wanted to check more precisely whether a common signal related to stephanodonty could be registered on the dental outline of both transgenic lines and species from the Apodemus and Stephanomys † lineages (excluding high-crowned Stephanomys † species, which are too derived; see Supplementary Table S3 and Supplementary Fig. S2 ). Therefore, we evaluated the impact of the morphological changes potentially associated to the addition of longitudinal crests on the M 1 overall shapes, especially on lateral cusps. Each species from the Apodemus and Stephanomys † lineages strongly diverge from Mus species and transgenic mice on the first axis of each analysis ( Fig. 4 ). This first-order signal corresponds to phylogenetic differences leading to idiosyncratic morphologies for each species. For instance, Mus and Progonomys † show different global shapes, nevertheless sharing an absent to weak stephanodont pattern. Stephanomys † species, especially the more recent forms, differ from the basal murine dental pattern in having enlarged cusps and much wider teeth [24] ( Fig. 4b ) and Apodemus bears an additional disto-lingual cusp. Nonetheless, a parallel trend possibly related to increased stephanodonty is observed on the second axis of each analysis ( Fig. 4 ). These shared modifications are related to variations of cusp size and location. For instance, a mesial location of the disto-vestibular cusp [t9] appears in Apodemus , Stephanomys † and transgenic species, and this is obviously related to the development of the garland. The more distal location of the mesio-lingual cusp [t1] allows the development of a mesio-lingual crest, a character that is similarly observed in transgenic mice and in Stephanomys † ( Fig. 4b ), but not in Apodemus ( Fig. 4a ). These stephanodont phenotypes are more pronounced in K14- Eda than in Edar Tg951/Tg951 ( Fig. 4 ), which agrees with the higher frequency of longitudinal crests in K14- Eda than in Edar Tg951/Tg951 ( Supplementary Fig. S1 ). 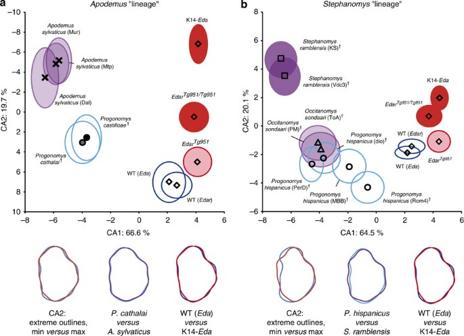Figure 4:Comparisons of M1outlines between stephanodont and transgenic forms. (a) Morphological space including the representatives of theApodemuslineage, and WT and transgenic mice. (b) Morphological space including theStephanomyslineage (early part), and WT and transgenic mice. Transgenic specimens with P4were not included here. Symbols represent the mean value of each sample and are associated to a species, whereas ellipses characterize the s.d. Open ellipses are associated to the absence of dental crest, filled ellipses with a clear colour are associated to basic to not fully developed stephanodont pattern, filled ellipses with a dark colour are associated to fully developed longitudinal crests. Dental outlines visualize shape changes associated to stephanodonty in several ways: extreme values along the second axis and superimposition of couples of non- or basic stephanodontversusfull stephanodont in the murine lineages and in transgenic lines (blue correspond to non- or basic stephanodont pattern, red and violet to more derived stephanodont pattern). †, extinct species; Dal, Dalhem (Belgium); Dio, Dionay (France); KS, Las Casiones (Spain); MBB, Masia del Barbo (Spain); Mtp, Montpellier (France); Mur, Murcia (Spain); PerD, Peralejos D (Spain); PM, Puente Minero (Spain); Rom4, La Roma 4 (Spain); ToA, Tortajada A (Spain); Vdc3, Valdecebro 3 (Spain). Figure 4: Comparisons of M 1 outlines between stephanodont and transgenic forms. ( a ) Morphological space including the representatives of the Apodemus lineage, and WT and transgenic mice. ( b ) Morphological space including the Stephanomys lineage (early part), and WT and transgenic mice. Transgenic specimens with P 4 were not included here. Symbols represent the mean value of each sample and are associated to a species, whereas ellipses characterize the s.d. Open ellipses are associated to the absence of dental crest, filled ellipses with a clear colour are associated to basic to not fully developed stephanodont pattern, filled ellipses with a dark colour are associated to fully developed longitudinal crests. Dental outlines visualize shape changes associated to stephanodonty in several ways: extreme values along the second axis and superimposition of couples of non- or basic stephanodont versus full stephanodont in the murine lineages and in transgenic lines (blue correspond to non- or basic stephanodont pattern, red and violet to more derived stephanodont pattern). †, extinct species; Dal, Dalhem (Belgium); Dio, Dionay (France); KS, Las Casiones (Spain); MBB, Masia del Barbo (Spain); Mtp, Montpellier (France); Mur, Murcia (Spain); PerD, Peralejos D (Spain); PM, Puente Minero (Spain); Rom4, La Roma 4 (Spain); ToA, Tortajada A (Spain); Vdc3, Valdecebro 3 (Spain). Full size image Abrasive and tough intakes in stephanodont species Dental microwear analyses revealed that all the investigated fossil and extant murine species display microwear patterns involving high number of fine scratches, pointing to a significant component of abrasive and tough intakes in the diet ( Fig. 5 and Supplementary Table S4 ). These particular physical properties may be related to the fragmentation and grinding down of herbaceous plants, such as grasses involving a high proportion of hard silica phytoliths, or of a co-ingestion of dust or grit frequently coating open environment plants [27] , [28] . Occitanomys † and Stephanomys † species have been expected to be grass eaters because of the dental enlargement trend coupled to the addition of longitudinal crests. However, Progonomys † species as well as the extinct Apodemus atavus † present a microwear pattern close to grass-dominated feeders ( Fig. 5 and Table 1 ), whereas they present a weak or complete garland, respectively. Consequently, the hypothesis of an ancestral omnivorous condition for both lineages is disputed ( Fig. 6 ). Results on extant Apodemus sylvaticus concur with previous observations of the stomach contents, indicating an omnivorous condition [29] , and emphasize its opportunistic behaviour because of the variations noticed from a forested to a slightly more open and dry area (that is, Belgium versus Spain; Table 1 and Supplementary Table S5 ). Species from the Stephanomys † lineage do not show any significant difference with grass-dominated feeders ( Fig. 5 and Table 1 ) and present the highest number of fine scratches (>19; Supplementary Table S4 ). 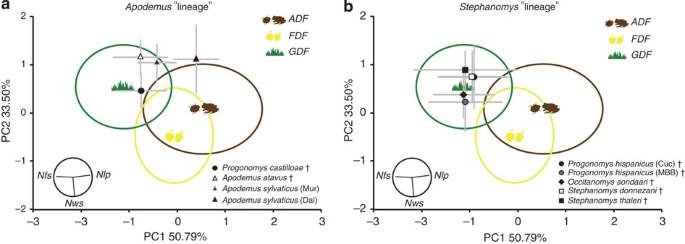Figure 5: Graphical comparisons of dental microwear patterns in stephanodont lineages. The principal component analysis was carried out on the tree variables (Nfs, number of fine scratches;Nws, number of wide scratches;Nlp, number of large pits). Dietary categories are based on the extant MUROIDEA database28. Cross-hair lines represent s.d. of the samples considered here, and coloured ellipses the s.d. of the three main ecological groups of the database. ADF, animal-dominated feeders; FDF, fruit-dominated feeders; GDF, grass-dominated feeders; †, extinct species; Cuc, Cucalón (Spain); Dal, Dalhem (Belgium); MBB, Masia del Barbo (Spain); Mur, Murcia (Spain). Figure 5: Graphical comparisons of dental microwear patterns in stephanodont lineages. The principal component analysis was carried out on the tree variables ( Nfs , number of fine scratches; Nws , number of wide scratches; Nlp , number of large pits). Dietary categories are based on the extant MUROIDEA database [28] . Cross-hair lines represent s.d. of the samples considered here, and coloured ellipses the s.d. of the three main ecological groups of the database. ADF, animal-dominated feeders; FDF, fruit-dominated feeders; GDF, grass-dominated feeders; †, extinct species; Cuc, Cucalón (Spain); Dal, Dalhem (Belgium); MBB, Masia del Barbo (Spain); Mur, Murcia (Spain). Full size image Table 1 Pairwise comparison tests performed on dental microwear data. 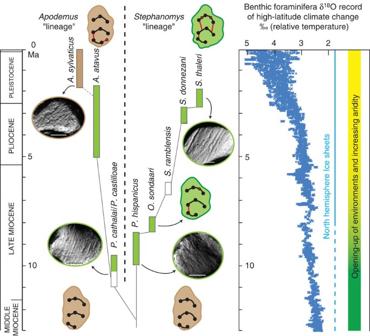Figure 6: Evolution of dietary habits in stephanodont lineages. Vertical boxes represent the stratigraphic range of each species with colour corresponding to the results of dental microwear analyses. Dental diagrams display hypothesized diet based on dental pattern (before the present study). Empty boxes represent species, which have only been studied for outline analyses. Brown signifies an omnivorous condition, and green an herbivorous condition with a significant abrasive and fibrous component (for example, grasses). Filled ellipses correspond to pictures of dental microwear (scale bar, 100 μm). The δ180 record characterizes the trend of high-latitude temperatures48,49, whereas the green and yellow box represent the gradient from closed and humid to open and arid environments is southwestern Europe derived from hypsodonty-based estimates of paleoprecipitations31. Full size table Figure 6: Evolution of dietary habits in stephanodont lineages. Vertical boxes represent the stratigraphic range of each species with colour corresponding to the results of dental microwear analyses. Dental diagrams display hypothesized diet based on dental pattern (before the present study). Empty boxes represent species, which have only been studied for outline analyses. Brown signifies an omnivorous condition, and green an herbivorous condition with a significant abrasive and fibrous component (for example, grasses). Filled ellipses correspond to pictures of dental microwear (scale bar, 100 μm). The δ 18 0 record characterizes the trend of high-latitude temperatures [48] , [49] , whereas the green and yellow box represent the gradient from closed and humid to open and arid environments is southwestern Europe derived from hypsodonty-based estimates of paleoprecipitations [31] . Full size image The morphological changes observed in Eda and Edar transgenic mice, which quantitatively affect the overall dental structure depending on the gene dosage, emphasize the potential involvement of the Eda pathway in the evolution of crests. In other words, our data show that longitudinal crests can originate from a relatively simple genetic and developmental change. Observations of global dental morphologies associated to quantification of dental outlines also show that the occurrence of longitudinal crests is coupled to the migration of certain cusps in upper molars of both the studied transgenic mice and stephanodont species. Shifts in cusp positions seem closely linked to the evolution of stephanodonty. Any differences in insertion of crests could be related to shapes inherited from diverse ancestral morphologies and to small variations in cusp locations. Indeed, crest insertions are also known to differ in some stephanodont species. For instance, the extinct Anthracomys † has the distal part of an anterior longitudinal crest connected to the central cusp instead of the lingual in first upper molars [8] . Taken together, details of cusp locations may constrain and bias the development and location of crests. Results of our dental microwear analyses support the idea that well-developed stephanodonty, together with swollen cusps, wide and high-crowned teeth, is likely an adaptation to grass consumption. This complex dental morphology, as very high-crowned teeth in some mammals, has been linked to the spread of grassland [30] , accompanied by the opening up of environments and aridification during the Late Miocene [31] ( Fig. 6 ). High-crowned teeth represent a genuine adaptation to abrasive matter, providing dental longevity in the face of rapid wear due to abrasive intakes. In all murine rodents, the cusp rows of each tooth simply slide in the gutter delimited by the cusp rows of the opposite tooth during antero-posterior chewing motions of the murine rasp [3] . In stephanodont species, the more the tooth is worn, the more the occlusal surface is enlarged without being extremely flat, which permits efficient shearing and grinding of food particles. The stephanodont pattern cannot be considered in itself as an adaptation to withstand intense wear induced by abrasive items, especially when it is not coupled to high-crown teeth. Longitudinal crests, as well as wider teeth [32] , can only enable a more efficient fragmentation and size reduction of herbaceous plants by increasing the occlusal surface, especially for highly fibrous plants such as grasses. Some extant African stephanodont species, such as Hybomys or Thallomys , do not frequently consume abrasive plants, whereas they occasionally ingest fibrous materials [4] . Therefore, the stephanodont pattern, especially in its basic form, should be interpreted as an efficient murine rasp necessary for processing fibrous rather than abrasive materials. A longstanding question in evolutionary biology research has been identifying factors promoting parallel and repeated morphological evolution. Basal murines, including Progonomys † species, had highly variable dental morphologies, including occasionally new crests, as in P. hispanicus † , or frequently supplementary cusps, as observed in the related P. clauzoni † (ref. 33 ). Our analyses show that comparable phenotypic variations can be observed in Edar heterozygous and homozygous transgenic mice regarding the occurrence of longitudinal crests. The Progonomys variants could have represented similarly simple developmental modifications with no immediate selective advantage, but which were later co-opted considering future environmental changes. In lineages leading to stephanodont species, the complete garland morphotype could have been positively selected as a means to enable a higher consumption of fibrous plants ( Fig. 6 ). Subsequently, directional selective events could have occurred in the Stephanomys † lineage, which tended to have wider and high-crowned teeth, coupled to a derived stage of stephanodonty. Their dental characteristics were likely related to diet specialization and the expansion of open environments involving grasslands, as suggested for Paraethomys † (refs 26 , 34 ). Interestingly, the highly specialized dentition of Stephanomys † did not enable this rodent to accommodate the frequent modifications of environments through the extreme climate variations of the Pleistocene interglacial–glacial periods, leading to its extinction 2 My ago [24] . In contrast, stabilizing selection could have prevailed in most other lineages having basic stephanodonty, such as Apodemus , which may have survived because of its broad tolerance to different environments and climates as shown by its present-day wide latitudinal distribution ranging from Scandinavia to North Africa [24] . The differences observed in the diet of A. sylvaticus between different regions (Belgium versus Spain) are another evidence for ecological flexibility of Apodemus . It is also possible that the basic stephanodonty represents an adaptively neutral phenotype evolving through pleiotropy, because natural selection operated on another, but genetically linked character. For example, a non-synonymous single-nucleotide variant, encoding EDAR370A, enhances the EDAR activity in humans [17] , [35] and underwent strong positive selection in Pleistocene East Asian human populations [35] , [36] . This variant also induces similar phenotypes in humans to those observed in Edar Tg951/Tg951 transgenic mice, such as thicker hair [37] and altered cutaneous glands [17] , [18] , which has recently been confirmed by the investigation of Edar370A knock-in mice [38] . In humans, the EDAR370A variant also contributes to the sinodont dental pattern characterized by enlarged teeth and shovelling of the incisors [39] , [40] . The dental phenotypes of East Asian humans and transgenic mice are likely to be dissimilar because of the differences in human and mouse dentitions, preventing the development of the stephanodont pattern in humans and the sinodont pattern in rodents. As Eda signalling affects multiple epithelial organs, it remains unclear what phenotypic characters have been under selection in individuals carrying the EDAR370A variant. Possibilities include hair and glands [18] , [37] , and the incisor shovelling may have been a byproduct of selection because of the unclear functional significance of this dental feature [39] . Interestingly, we note that the basic stephanodont murine, Apodemus sylvaticus , has significantly thicker fur than Mus musculus [41] . However, the pleiotropic effects of Eda signaling in extant murine species remains to be investigated. In conclusion, we have demonstrated that the longitudinal crests mimicking the stephanodont pattern can be easily obtained in the mouse with only minor genetic modifications. This relatively simple developmental modification can explain the multiple parallel appearances of this phenotype over the course of murine evolution. Whereas in advanced stages, stephanodonty is clearly associated with dietary adaptations to tough foods, basic stephanodonty may have also been selectively neutral, and potentially arisen through pleiotropy following positive selection upon a non-dental trait. This work demonstrates that integrating the study of developmental mechanisms together with that of function of novel morphologies aids in the evaluation of scenarios underlying their evolutionary origin. Dental morphology We studied the dental morphology of transgenic lines corresponding to FVB/N mice ( Mus musculus ) with increased Eda expression under the heterologous keratin-14 promoter [22] and with increased copy number of Edar under its endogenous regulatory elements [17] . For the K14- Eda mice all procedures were performed under the University of Helsinki and governmental licences, and for the Edar Tg951 line all procedures were performed under a UK Government Home Office licence. The statistical sets of specimens encompass homozygous 29 K14- Eda , 30 homozygous Edar Tg951/Tg951 and 10 heterozygous Edar Tg951 mice compared with two sets of six and nine strain-matched controls (WT). Both males and females older than 1 month and having a fully erupted dentition were studied. Dental rows were digitized using a stereomicroscope (Leica M165C) connected to a spot CCD camera (Leica DFC420) and then measured using the LAS Core software (Leica). Imaging High-quality images of homozygous transgenic and WT mice dentitions were obtained at the European Synchrotron Radiation Facility (Grenoble, France), beamline ID19, with monochromatic X-ray beams at energy of 25 keV and using a cubic voxel of 5.06 μm. This method has been proven to be very efficient for very precise imaging of small elements [42] , including rodent teeth [43] . Other dentitions were imaged using a GE phoenix nanotom 180 at energy of 100 keV with a cubic voxel of 2.73 or 2.51 μm for heterozygous transgenic mice, of 3.48 or 4.95 μm for Apodemus sylvaticus , and of 5.20 μm for Stephanomys donnezani † . Three-dimensional renderings were then performed using VGStudio Max 2.0 software. Outline analyses Quantifications of two-dimensional dental outline of M 1 were performed on transgenic, WT mice and a database involving extant and extinct murine rodents [24] , [26] ( Supplementary Table S3 ), most of them being stephanodont to various degrees. Dental outline analysis was performed by means of radial Fourier transform [44] . This method allows the description of complex outlines approximating them by a sum of trigonometric functions of decreasing wavelength (that is, harmonics). We retained the first nine harmonics for M 1 , which represent an efficient compromise between measurement error and information content for these murine molars [34] . Each harmonic is described by two coefficients. As a result, the 18 coefficients were used as multivariate shape variables to perform canonical analyses, which permit visualization of the main patterns of morphological differentiation between groups. Dental microwear analyses Dental microwear patterns were investigated by using transmitted light stereomicroscopy with a protocol adapted to the small dentition of rodents [45] . This method permits reconstruction of the last diet items ingested by an animal before death [46] , [47] . Seven extant and extinct species from Stephanomys † and Apodemus lineages were compared with a database (that is, MUROIDEA) based on extant rodents [28] ( Supplementary Table S3 ). A principal component analysis was performed on three variables, the numbers of fine scratches ( Nfs ), wide scratches ( Nws ) and large pits ( Nlp ), used to infer the main dietary component of stephanodont species. Multiple mean comparison tests, the Fischer’s least significant difference test and the more conservative Tukey’s honestly significant difference test were used to determine the source of variations between dietary groups and stephanodont species. How to cite this article: Gomes Rodrigues, H. et al. Roles of dental development and adaptation in rodent evolution. Nat. Commun. 4:2504 doi: 10.1038/ncomms3504 (2013).